Hypothalamic S1P/S1PR1 axis controls energy homeostasis Sphingosine 1-phosphate receptor 1 (S1PR1) is a G-protein-coupled receptor for sphingosine-1-phosphate (S1P) that has a role in many physiological and pathophysiological processes. Here we show that the S1P/S1PR1 signalling pathway in hypothalamic neurons regulates energy homeostasis in rodents. We demonstrate that S1PR1 protein is highly enriched in hypothalamic POMC neurons of rats. Intracerebroventricular injections of the bioactive lipid, S1P, reduce food consumption and increase rat energy expenditure through persistent activation of STAT3 and the melanocortin system. Similarly, the selective disruption of hypothalamic S1PR1 increases food intake and reduces the respiratory exchange ratio. We further show that STAT3 controls S1PR1 expression in neurons via a positive feedback mechanism. Interestingly, several models of obesity and cancer anorexia display an imbalance of hypothalamic S1P/S1PR1/STAT3 axis, whereas pharmacological intervention ameliorates these phenotypes. Taken together, our data demonstrate that the neuronal S1P/S1PR1/STAT3 signalling axis plays a critical role in the control of energy homeostasis in rats. The hypothalamus plays an important role in the regulation of energy homeostasis controlling feeding behaviour and energy metabolism in mammals [1] . Body weight and appetite control are complex and incompletely characterized. It has been postulated that central mechanisms disturbance can lead to hyperfagia or anorexia. In this context, Janus kinase/signal transducer and activator of transcription (Jak/STAT) signalling plays a fine tune in the control of anorexigenic and thermogenic signal on hormonal [2] , [3] or inflammatory stimulus [4] , [5] , [6] . The disturbance in the hypothalamic Jak2/STAT3 signalling results in anomalous neurotransmitters production, generating abnormal anorexigenic and thermogenic response, and favouring body mass gain or severe weight loss [5] , [7] , [8] , [9] , [10] . Thus, alternative strategies to control Jak/STAT cascade activation in the hypothalamus could be considered as potential therapeutic targets to maintain the energy homeostasis during abnormal feeding behaviour, such as hyperphagia and anorexia. Recently, a class of sphingosine 1-phosphate receptors (S1PRs) has been implicated in the control of Jak2/STAT3 signalling [11] , [12] , [13] , [14] . S1PRs family is comprises five (1–5) specific G-protein-coupled receptors that activate diverse downstream signalling pathways in response to the common sphingosine-1-phosphate (S1P) [15] . The lysophospholipid, S1P, is a circulating bioactive lipid metabolite formed by phosphorylation of sphingosine, in a reaction catalysed by sphingosine kinase, SPHK1 and 2 (ref. 16 ). S1P/S1PRs axis plays a important role in the control of cardioprotection [11] , intestinal inflammation [12] , satellite cell activation [17] and tumour cells progression [13] through the persistent STAT3 activation. However, the role of hypothalamic S1P/S1PR1/STAT3 axis in the control of the energy homeostasis was not reported. Here we combined the physiological, pharmacological and genetic approaches, and transcriptome analysis to investigate the participation of hypothalamic S1P/S1PR1 axis in the control of anorexigenic signals, food consumption and energy expenditure in rodents. In addition, we examined the role of neuronal S1P/S1PR1/STAT3 signalling in distinct conditions of abnormal feeding behaviour, including obesity and cancer-induced anorexia. Characterization of hypothalamic S1PR1 We sought to determine the role of S1PR1 in hypothalamic neurons in the control of the energy homeostasis. First, we evaluate the distribution of S1PR1 in different tissues of normal rats and observed that the S1PR1 protein was highly enriched in the hypothalamus, when compared with peripheral tissues, such as the heart, liver, skeletal muscle and adipose tissues ( Fig. 1a ). Thereafter, we examine the S1PR1 distribution pattern in the hypothalamus using the micro dissection of hypothalamic nuclei. This technique revealed that S1PR1 is expressed predominantly in the arcuate and ventromedial/dorsomedial nuclei in the hypothalamus and low protein levels were found in paraventricular (PVN) nucleus and in lateral hypothalamus ( Fig. 1b ). These data were confirmed by immunostaining assay ( Fig. 1c , left panel). We also employed the double staining and observed that S1PR1 is stained predominantly in anorexigenic (pro-opiomelanocortin (POMC)), but not in orexigenic (neuropeptide Y (NPY)) neurons in the arcuate nucleus ( Fig. 1c ). We noted that S1PR1 is stained in the neurons but is barely stained in non-neuronal cells (such as astrocytes) in the arcuate nucleus ( Supplementary Fig. 1A ). We also monitored the S1PR1 expression in other regions of the brain, including forebrain, midbrain and hindbrain, and high levels of S1PR1 were also found in midbrain of rats ( Supplementary Fig. 1B ). 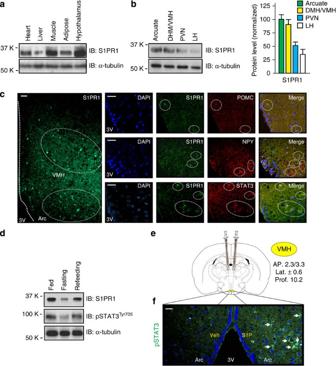Figure 1: Characterization of S1PR1 in the hypothalamus of rats. Western blottings show (a) S1PR1 protein levels in different tissues of control rats (n=6). (b) S1PR1 protein levels in the arcuate (Arc), dorsomedial/vetromedial (DMH/VMH), PVN nucleus and in the lateral hypothalamus (LH) of control rats (n=6). Bars represent the mean±s.e.m. (c) Single and double immunostaining was performed to evaluate the co-localization of S1PR1 (green) with POMC, NPY and STAT3 (red) in the arcuate nuclei of rats, with × 50 magnification (left panel) or × 200 magnification (scale bar, 20 μm). (d) Western blotting shows the S1PR1 protein levels and STAT3 tyrosine phosphorylation in hypothalamic samples of rats at 12 h of fasting and after 6 h of refeeding (n=5). (e) A schematic representation showing the localization of S1P injection. S1P was injected into the VMH of rats (coordinates 2.3/3.3 mm posterior to the bregma, ±0.6 mm lateral to midline and 10.2 mm below the surface of the skull). (f) Single immunostaining was performed to evaluate STAT3 tyrosine phosphorylation (green) in the hypothalamus of rats 30 min after vehicle (left) or S1P 50 ng (right) injections in the same rat, with × 100 magnification (scale bar, 20 μm). Figure 1: Characterization of S1PR1 in the hypothalamus of rats. Western blottings show ( a ) S1PR1 protein levels in different tissues of control rats ( n =6). ( b ) S1PR1 protein levels in the arcuate (Arc), dorsomedial/vetromedial (DMH/VMH), PVN nucleus and in the lateral hypothalamus (LH) of control rats ( n =6). Bars represent the mean±s.e.m. ( c ) Single and double immunostaining was performed to evaluate the co-localization of S1PR1 (green) with POMC, NPY and STAT3 (red) in the arcuate nuclei of rats, with × 50 magnification (left panel) or × 200 magnification (scale bar, 20 μm). ( d ) Western blotting shows the S1PR1 protein levels and STAT3 tyrosine phosphorylation in hypothalamic samples of rats at 12 h of fasting and after 6 h of refeeding ( n =5). ( e ) A schematic representation showing the localization of S1P injection. S1P was injected into the VMH of rats (coordinates 2.3/3.3 mm posterior to the bregma, ±0.6 mm lateral to midline and 10.2 mm below the surface of the skull). ( f ) Single immunostaining was performed to evaluate STAT3 tyrosine phosphorylation (green) in the hypothalamus of rats 30 min after vehicle (left) or S1P 50 ng (right) injections in the same rat, with × 100 magnification (scale bar, 20 μm). Full size image Once S1PR1 is localized in hypothalamic nuclei and in neurons specialized in the control of energy homeostasis, we sought to determine whether the physiological nutritional status modulates the hypothalamic S1PR1 expression. We observed that 12 h of fasting was sufficient to reduce S1PR1 protein level in the hypothalamus of control rats by about 60%, whereas the refeeding period (6 h) restored the protein levels of this receptor ( Fig. 1d ). In addition, hypothalamic STAT3 tyrosine phosphorylation accompanied the pattern of S1PR1 protein levels in the fasting/refeeding experiment ( Fig. 1d , middle panel). After these results, we hypothesized that neuronal S1PR1 could be involved in the control of the energy homeostasis through the positive cross-talk mechanism, involving Jak/STAT3 cascade in neurons, as observed in other cell types [11] , [12] , [13] , [14] , [17] . Next, we examined the relationship between the S1PR1 and Jak/STAT signalling in the hypothalamus. We detected that most neurons expressing S1PR1 in the arcuate nucleus were shown to possess STAT3 in control rats, suggesting a possible interaction between these molecules ( Fig. 1c , lower panels). To determine whether S1PR1 activates hypothalamic STAT3, we next carried out a bilateral cannulation to access the ventromedial hypothalamus (VMH; Supplementary Fig. 1C ), and then used the endogenous S1PR1 activator, S1P (50 ng), into one side of the VMH and vehicle into the other side of the VMH in the same rat ( Fig. 1e ), as previously described [18] . Interestingly, S1P, but not vehicle, induced tyrosine phosphorylation of STAT3 in the hypothalamus of control rats ( Fig. 1f ). Collectively, these data indicate that the hypothalamic S1PR1 is localized in the mediobasal of the hypothalamus in neurons specialized in the control of energy homeostasis, and that S1PR1 activation increases the STAT3 activity in the hypothalamus of rats. Central S1P/S1PR1 controls energy homeostasis Thereafter, we evaluate the effects of S1PR1 activator, S1P, in the control of food intake and energy expenditure in rodents. We performed an acute injection of S1P in the third ventricle of rats in different doses (2 and 50 ng) and monitored the food consumption during 4 and 12 h. S1P reduced the food intake in a dose-dependent manner ( Fig. 2a ). To evaluate the possibility that the anorectic effect of S1P was caused by an aversive effect, we measured taste reactivity after acute intracerebroventricular (ICV) S1P injection. The total numbers of hedonic, neutral and aversive reactions remained unchanged ( Supplementary Fig. 2A ). We also performed chronic (3 days) of ICV S1P (50 ng) injections and we observed a consistent anorexigenic effect during 3 consecutive days in control rats; on the other hand, after these injections, these animals rapidly returned to the baseline of food intake, in a similar manner as observed in the pair-feeding group ( Supplementary Fig. 2B ). These data demonstrated that S1P ICV injection does not evoke a taste aversion or toxic effect. 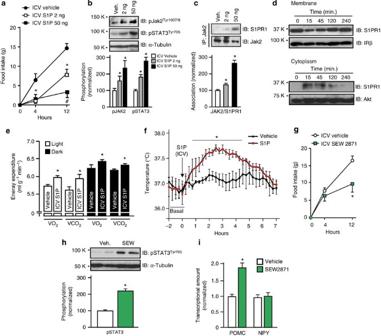Figure 2: Neuronal S1PR1 activation induces anorexigenic and thermogenic response. (a) Determination of food consumption after ICV injection of S1P (2 or 50 ng) in control rats (n=8). (b) Western blottings show S1P-induced Jak2tyr1007/1008and STAT3tyr705phosphorylation in hypothalamic samples of Wistar rats 30 min after S1P injections (n=6). (c) Immunoprecipitation assay was performed to evaluate S1PR1/Jak2 association 30 min after S1P injections (n=6). (d) Subcellular fractionation was performed to evaluate S1PR1 expression in membrane and cytoplasm of samples obtained from control rats injected with S1P (50 ng). (e) Oxygen consumption/carbon dioxide production after single injection of S1P into the third ventricle of control rats. (f) Evaluation of the body temperature after acute ICV injection of S1P (50 ng) in control rats (n=5). (g) Determination of food consumption after ICV injection of SEW2871 (50 nM) in control rats (n=6). (h) Western blotting shows SEW-induced STAT3tyr705phosphorylation in hypothalamic samples of Wistar rats 30 min after SEW injection (n=4). (i) POMC and NPY mRNA were examined using real-time PCR assay 9 h after IICV SEW2871 (50 nM) injection (n=8). Data were expressed by using mean±s.e.m.*P<0.05 versus vehicle and #P<0.05 versus S1P 2 ng. One-way analysis of variance was used for statistical analysis in thea–cand unpairedt-test was used ine–i. Figure 2: Neuronal S1PR1 activation induces anorexigenic and thermogenic response. ( a ) Determination of food consumption after ICV injection of S1P (2 or 50 ng) in control rats ( n =8). ( b ) Western blottings show S1P-induced Jak2 tyr1007/1008 and STAT3 tyr705 phosphorylation in hypothalamic samples of Wistar rats 30 min after S1P injections ( n =6). ( c ) Immunoprecipitation assay was performed to evaluate S1PR1/Jak2 association 30 min after S1P injections ( n =6). ( d ) Subcellular fractionation was performed to evaluate S1PR1 expression in membrane and cytoplasm of samples obtained from control rats injected with S1P (50 ng). ( e ) Oxygen consumption/carbon dioxide production after single injection of S1P into the third ventricle of control rats. ( f ) Evaluation of the body temperature after acute ICV injection of S1P (50 ng) in control rats ( n =5). ( g ) Determination of food consumption after ICV injection of SEW2871 (50 nM) in control rats ( n =6). ( h ) Western blotting shows SEW-induced STAT3 tyr705 phosphorylation in hypothalamic samples of Wistar rats 30 min after SEW injection ( n =4). ( i ) POMC and NPY mRNA were examined using real-time PCR assay 9 h after IICV SEW2871 (50 nM) injection ( n =8). Data were expressed by using mean±s.e.m. * P <0.05 versus vehicle and # P <0.05 versus S1P 2 ng. One-way analysis of variance was used for statistical analysis in the a – c and unpaired t -test was used in e – i . Full size image Western blotting analysis confirmed that S1P increased Jak2 and STAT3 tyrosine phosphorylation in the hypothalamus in a dose-dependent manner ( Fig. 2b ). To investigate whether S1PR1 activates directly the leptin signal transduction, we carried out immunoprecipitation assay to evaluate the S1PR1/Jak2 association. Our experiments revealed that acute ICV injection of S1P promoted the S1PR1/Jak2 association in the hypothalamic tissue in a dose-dependent manner ( Fig. 2c ). However, acute microinjection of S1P did not change the insulin receptor substrate 1 (IRS1) and Akt phosphorylation in the hypothalamus ( Supplementary Fig. 2C ). It has been proposed that S1P mediates its biological effects inducing S1PR1 internalization and subsequent degradation [15] , [19] . To address the efficacy of S1P injection on S1PR1 activation, we examine the subcellular expression of S1PR1 after S1P (50 ng) ICV injection. We observed the downregulation of S1PR1 in the membrane of the cells between 15 and 45 min after S1P stimulus; this phenomenon was accompanied by transitory cytoplasmic S1PR1 accumulation, suggesting that S1P induced activation and internalization of S1PR1 in hypothalamic cells ( Fig. 2d ). We also monitored the energy expenditure and body temperature after acute S1P (50 ng) injection. The ICV S1P injection increased the energy expenditure in rats, increasing the O 2 consumption and CO 2 production, in both, light and dark periods ( Fig. 2e ), without any change in the physical activity pattern ( Supplementary Fig. 2D ). ICV injection of S1P also promoted the elevation of body temperature when compared with vehicle ( Fig. 2f ). These data demonstrated that hypothalamic S1PR1 stimulation induced a potent anorexigenic and thermogenic action. Although S1P is considered the main endogenous S1PR1 activator, this molecule is able to activate other S1PRs [20] . Thus, we performed an acute microinjection of specific S1PR1 activator (SEW2871) into the third ventricle of rats. We observed that SEW2871 (50 nM) reproduced the effects of S1P, reducing the food intake ( Fig. 2g ) and activating the leptin signalling ( Fig. 2h ). Consistent with the role of the hypothalamic S1PR1 activation in the control of food consumption and on STAT3 activation, we observed that acute SEW2871 injection into the third ventricle of rats modulates the expression of neuropeptides involved in the food intake and energy expenditure control. SEW2871 increased POMC messenger RNA without changing NPY mRNA levels, when compared with vehicle injection ( Fig. 2i ). Next, we evaluate the impact of intraperitoneal S1P injection (100 ng) on food intake and on energy expenditure in mice. Interestingly, acute intraperitoneal injection of S1P reduced the food consumption and promoted a discrete but significant increase in energy expenditure ( Supplementary Fig. 2E,F ). No statistical difference in body temperature was observed in C57BL6/J mice after acute intraperitoneal injection of S1P (peak of temperature; Veh. 37.3±0.5 °C versus S1P 37.5±0.8 °C). S1PR1 requires the leptin signalling and melanocortin system It has been demonstrated that Jak2/STAT3 signalling activators, including interleukin-6, promotes a transient STAT3 activation, while S1PR1 induces a persistent STAT3 phosphorylation [13] . Based on this information, we suspected that S1P could induce a potent anorexigenic effect through the persistent STAT3 activation. To address this question, we performed a time-course study to examine STAT3 phosphorylation on acute leptin or S1P ICV injections. The western blotting analysis revealed that ICV infusion of leptin promoted a transient effect on STAT3 phosphorylation. Leptin increased the tyrosine phosphorylation of STAT3 after 15 and 30 min, returning at the basal levels after 60 min ( Fig. 3a,b ). Notably, the ICV infusion of S1P promoted potent and persistent phosphorylation of this molecule, increasing STAT3 phosphorylation after 5 min and peaking at 120 min later ( Fig. 3a,b ). We also monitored the food consumption after acute leptin or S1P ICV injection in control rats and we observed that S1P promoted a potent and persistent anorexigenic effect when compared with leptin ( Fig. 3c ). 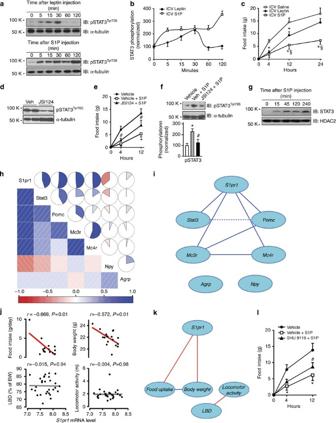Figure 3: S1PR1 requires STAT3 activation to induce anorexia. (a) Western blottings show leptin-induced STAT3 phosphorylation (upper panel) and S1P-induced STAT3 phosphorylation (lower panel) after ICV stimulation (n=4 in each point). (b) Representation of STAT3 phosphorylation pattern after leptin or S1P ICV injections. (c) Determination of food consumption after ICV injection of saline (2 μl), leptin (10−6M) or S1P (50 ng) in control rats (n=10). (d) Western blotting shows the effects of JSI124 (50 μM) on STAT3 phosphorylation in the hypothalamus (n=4). (e) Food intake evaluation after vehicle (2 μl), S1P (50 ng) and JSI124 (50 μM) plus S1P injection. (f) Western blotting shows the effects of JSI124 (50 μM) on S1P-induced STAT3 phosphorylation in the hypothalamus (n=4). (g) Nuclear STAT3 translocation after ICV injection of S1P (50 ng) (n=3, in each point). (h) Correlation matrices (left lower triangle) and pie graphs (right upper triangle) showing correlations amongS1pr1,Stat3,Pomc,Mc3r,Mc4r,NpyandAgrpin the hypothalamus of the BXD inbred family (n=33, GSE36674). The depth of the shading at the correlation matrices indicates the magnitude of the correlation. Positive and negative correlations are represented in blue and red, respectively. The pie graphs are filled in proportion to the Pearson’s coefficient values, clockwise for positive correlations (in blue) and anti-clockwise for negative correlations (in red). (i) Interaction network showing correlations of indicated genes. Positive Pearson’s correlation coefficients are represented by blue solid (r=0.5–1.0) and dashed line (r=0.4–0.5). (j) Correlation plots between hypothalamicS1pr1and each indicated phenotype (n=10 to 29). Pearson’s coefficient values were used to analyse correlations, and Pearson’srandP-values are indicated. (k) Interaction network showing correlations between hypothalamicS1pr1and each indicated phenotype. Positive Pearson’s correlation coefficients are represented by blue and red lines (r=0.5–1.0). (l) Food consumption evaluation was performed after vehicle (2 μl), S1P (50 ng) and SHU9119 (1 mmol) plus S1P injection (n=5). Data were expressed by using mean±s.e.m. *P<0.05 versus vehicle, §P<0.05 versus leptin group and #P<0.05 versus vehicle plus S1P. One-way analysis of variance and Bonferroni post test were performed ine,fandl. Figure 3: S1PR1 requires STAT3 activation to induce anorexia. ( a ) Western blottings show leptin-induced STAT3 phosphorylation (upper panel) and S1P-induced STAT3 phosphorylation (lower panel) after ICV stimulation ( n =4 in each point). ( b ) Representation of STAT3 phosphorylation pattern after leptin or S1P ICV injections. ( c ) Determination of food consumption after ICV injection of saline (2 μl), leptin (10 −6 M) or S1P (50 ng) in control rats ( n =10). ( d ) Western blotting shows the effects of JSI124 (50 μM) on STAT3 phosphorylation in the hypothalamus ( n =4). ( e ) Food intake evaluation after vehicle (2 μl), S1P (50 ng) and JSI124 (50 μM) plus S1P injection. ( f ) Western blotting shows the effects of JSI124 (50 μM) on S1P-induced STAT3 phosphorylation in the hypothalamus ( n =4). ( g ) Nuclear STAT3 translocation after ICV injection of S1P (50 ng) ( n =3, in each point). ( h ) Correlation matrices (left lower triangle) and pie graphs (right upper triangle) showing correlations among S1pr1 , Stat3 , Pomc , Mc3r , Mc4r , Npy and Agrp in the hypothalamus of the BXD inbred family ( n =33, GSE36674). The depth of the shading at the correlation matrices indicates the magnitude of the correlation. Positive and negative correlations are represented in blue and red, respectively. The pie graphs are filled in proportion to the Pearson’s coefficient values, clockwise for positive correlations (in blue) and anti-clockwise for negative correlations (in red). ( i ) Interaction network showing correlations of indicated genes. Positive Pearson’s correlation coefficients are represented by blue solid ( r =0.5–1.0) and dashed line ( r =0.4–0.5). ( j ) Correlation plots between hypothalamic S1pr1 and each indicated phenotype ( n =10 to 29). Pearson’s coefficient values were used to analyse correlations, and Pearson’s r and P -values are indicated. ( k ) Interaction network showing correlations between hypothalamic S1pr1 and each indicated phenotype. Positive Pearson’s correlation coefficients are represented by blue and red lines ( r =0.5–1.0). ( l ) Food consumption evaluation was performed after vehicle (2 μl), S1P (50 ng) and SHU9119 (1 mmol) plus S1P injection ( n =5). Data were expressed by using mean±s.e.m. * P <0.05 versus vehicle, § P <0.05 versus leptin group and # P <0.05 versus vehicle plus S1P. One-way analysis of variance and Bonferroni post test were performed in e , f and l . Full size image To confirm whether S1PR1 anorexigenic action depends on the Jak2 and STAT3 signalling, we used the pretreatment with the inhibitor of STAT3, JSI124, before the S1P injection. To test the efficacy of JSI124 in the hypothalamus, we performed an acute injection using 50 μM into the third ventricle of control animals. Western blot analysis showed that JSI124 reduced STAT3 tyrosine phosphorylation, when compared with vehicle injection ( Fig. 3d ). Interestingly, the JSI124 pretreatment, 30 min before S1P ICV injection, was sufficient to block, at least in part, the anorexigenic action of S1P injection ( Fig. 3e ) and reduced the S1P-induced STAT3 phosphorylation in the hypothalamus ( Fig. 3f ). Acutely, ICV JSI124 alone did not change the food consumption (Veh. 13.8±1.2 g versus JSI124 12.6±2.3 g). Accumulating number of studies have demonstrated that hypothalamic STAT3 tyrosine 705 phosphorylation precedes STAT3 DNA binding, promoting transcriptional activation of the POMC promoter, induced by anorexigenic factors, including leptin [2] , [21] , [22] , [23] or cytokines [24] , [25] , [26] . Thus, we evaluated the STAT3 nuclear translocation after S1P ICV injection in control rats. The time-course study revealed that S1P (50 ng) induced a rapid and persistent STAT3 nuclear accumulation ( Fig. 3g ). To confirm our experimental findings, we performed a bioinformatics analysis using the BXD murine reference panel for multiscalar integration of traits previously published [27] . The transcriptome data from the hypothalamus revealed that S1pr1 mRNA levels strongly correlated with the expression of Pomc in the hypothalamus of BXD inbred strains ( n =33). Furthermore, we also found a strong positive correlation among hypothalamic S1pr1 mRNA, and Mc3r and Mc4r , without correlation between S1pr1 , and Agrp and Npy levels. ( Fig. 3h,i ). Not surprisingly, hypothalamic S1pr1 expression has a strong negative correlation with food intake and body weight but not with locomotor activity and lean body mass ( Fig. 3j,k ). These data are in accordance with our experimental data and suggest that the anorexigenic S1PR1 signal could be projected to the secondary neurons, involving the melanocortin system. To confirm the role of S1PR1 on melanocortin system, we performed the ICV injection of a potent melanocortin MC3 and MC4 receptor antagonist, SHU9119 (1.0 mM), in control rats. This experiment revealed that SHU9119 pretreatment partially prevented the anorexigenic effects of S1P ICV injection ( Fig. 3l ). These data indicate that an anorexigenic effect of hypothalamic S1P/S1PR1 axis requires, at least in part, the STAT3 activation and the melanocortin system. Hypothalamic S1PR1 disruption affects the energy homeostasis Next, we examined the effects of specific hypothalamic S1PR1 knockdown using the small interfering RNAs (siRNAs) in vivo , as previously described [28] , [29] . The siRNA against S1PR1 was complexed with JetSI lipids and administered bilaterally into the mediobasal hypothalamus (MBH) of intact mice. To access the MBH of mice, we performed an acute bilateral injection, as represented in the Fig. 4a . The time-course study revealed that S1PR1 siRNA injection promoted a transient reduction S1PR1 protein levels in the VMH/ dorsomedial hypothalamus (DMH), whereas the efficacy of the siRNA was about 60% in the first 24 h ( Fig. 4b ). The siRNA reduced S1PR1 protein level in the arcuate nucleus, without change S1PR1 protein level in other brain areas, including, forebrain, midbrain and hindbrain ( Fig. 4c ). Interestingly, the hyperphagic response was observed only during the transient disruption of S1PR1 MBH of mice ( Fig. 4d ). The hyperphagia persisted until 36 h after S1PR1 siRNA injection ( Fig. 4e ). Consistent with the downregulation of hypothalamic S1PR1, low levels of STAT3 phosphorylation were observed in mice under fed condition ( Fig. 4f ). No difference in the total body weight was observed 48 h after S1PR1 siRNA injection (Scramble 26.3±0.6 g versus 26.7±0.7 g). 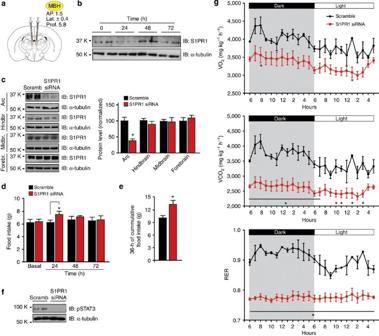Figure 4: Effect of S1PR1 siRNA on food consumption and energy expenditure. (a) A schematic representation showing the localization of S1PR1 siRNA injection into the MBH of mice (coordinates of 1.5 mm posterior to the bregma, 5.8 mm below the surface of the skull and 0.4 mm lateral to midline). (b) Time-course of S1PR1 protein levels in VMH/DMH after S1PR1 siRNA injection in mice. (c) S1PR1 protein levels in different brain regions. (d) Daily food consumption after S1PR1 siRNA injection in mice (n=6). (e) Thirty-six hours of cumulative food intake (n=6). (f) Western blotting shows the effects of S1PR1 siRNA on STAT3 phosphorylation in the hypothalamus in mice fed on chow diet (n=4). (g) Oxygen consumption, carbon dioxide production and respiratory exchange ratio during 24 h after S1PR1 siRNA injection (n=6). Data were expressed by using mean±s.e.m.*P<0.05 versus scramble (Student’st-test). Figure 4: Effect of S1PR1 siRNA on food consumption and energy expenditure. ( a ) A schematic representation showing the localization of S1PR1 siRNA injection into the MBH of mice (coordinates of 1.5 mm posterior to the bregma, 5.8 mm below the surface of the skull and 0.4 mm lateral to midline). ( b ) Time-course of S1PR1 protein levels in VMH/DMH after S1PR1 siRNA injection in mice. ( c ) S1PR1 protein levels in different brain regions. ( d ) Daily food consumption after S1PR1 siRNA injection in mice ( n =6). ( e ) Thirty-six hours of cumulative food intake ( n =6). ( f ) Western blotting shows the effects of S1PR1 siRNA on STAT3 phosphorylation in the hypothalamus in mice fed on chow diet ( n =4). ( g ) Oxygen consumption, carbon dioxide production and respiratory exchange ratio during 24 h after S1PR1 siRNA injection ( n =6). Data were expressed by using mean±s.e.m. * P <0.05 versus scramble (Student’s t -test). Full size image We also measured the energy expenditure during 24 h after S1PR1 siRNA injection in MBH of mice. These mice displayed reduction in the energy expenditure, as demonstrated by the low levels of VCO 2 production and respiratory exchange ratio ( Fig. 4g ). Taken together, these data demonstrated that transient S1PR1 disruption in discrete hypothalamic nucleus alters the energy balance in mice. STAT3 controls the hypothalamic S1PR1 protein levels The transcriptome data from hypothalamus of BXD mice demonstrated a strong positive correlation between Stat3 and S1pr1 levels ( Fig. 3h,i ). In accordance with this data, it has been demonstrated that STAT3 directly binds to the S1pr1 promoter, increasing the S1PR1 mRNA levels in tumour cells [13] . To address whether STAT3 activation modulates S1PR1 protein levels in neurons, we employed the cell culture system using neuronal GT1-7 cells treated with leptin. We carried out a time-course study and observed that leptin (40 μmol l −1 ) increased S1PR1 protein levels in GT1-7 cells in a time-dependent manner ( Fig. 5a ). Next, we used STAT3 siRNA in GT1-7 cells ( Fig. 5b ) to evaluate the requirement of STAT3 on leptin-induced S1PR1 expression. We observed that leptin failed to increase S1PR1 protein levels in GT1-7 cells transfected with STAT3 siRNA ( Fig. 5c ). 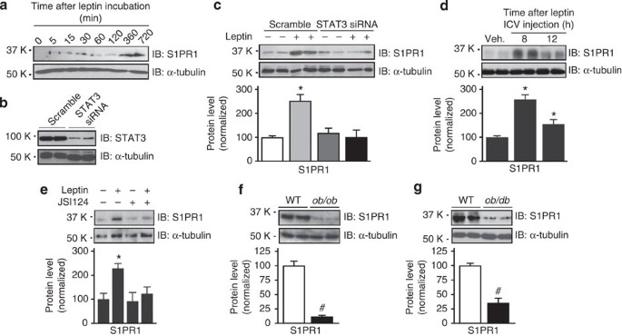Figure 5: STAT3 controls S1PR1 protein levels in neurons. Western blottings show (a) S1PR1 protein levels in GT1-7 cells after leptin (40 μmol l−1) incubation, performed in three independent experiments. (b) Effect of STAT3 siRNA transfection on STAT3 protein levels in GT1-7 cells. (c) Effect of leptin (40 μmol l−1) incubation on S1PR1 protein levels in GT1-7 cells transfected with STAT3 siRNA. (d) Effect of leptin on S1PR1 protein levels in the hypothalamus of control rats (n=4). Hypothalamic samples were obtained 8 and 12 h after acute leptin (10−6M) injection. (e) S1PR1 protein levels in control rats injected with saline (2 μl), leptin (10−6M) or JSI124 plus leptin. Hypothalamic samples were obtained 8 h after leptin injection (n=4). (f) Evaluation of S1PR1 protein levels on the hypothalamus ofob/obmice and (g)db/dbmice, and C57BL6/J (n=4). Data were expressed by using mean±s.e.m. *P<0.05 versus vehicle and#P<0.05 versus wild-type (Student’st-test). Figure 5: STAT3 controls S1PR1 protein levels in neurons. Western blottings show ( a ) S1PR1 protein levels in GT1-7 cells after leptin (40 μmol l −1 ) incubation, performed in three independent experiments. ( b ) Effect of STAT3 siRNA transfection on STAT3 protein levels in GT1-7 cells. ( c ) Effect of leptin (40 μmol l −1 ) incubation on S1PR1 protein levels in GT1-7 cells transfected with STAT3 siRNA. ( d ) Effect of leptin on S1PR1 protein levels in the hypothalamus of control rats ( n =4). Hypothalamic samples were obtained 8 and 12 h after acute leptin (10 −6 M) injection. ( e ) S1PR1 protein levels in control rats injected with saline (2 μl), leptin (10 −6 M) or JSI124 plus leptin. Hypothalamic samples were obtained 8 h after leptin injection ( n =4). ( f ) Evaluation of S1PR1 protein levels on the hypothalamus of ob/ob mice and ( g ) db/db mice, and C57BL6/J ( n =4). Data were expressed by using mean±s.e.m. * P <0.05 versus vehicle and # P <0.05 versus wild-type (Student’s t -test). Full size image We then evaluated the effects of leptin in the control of S1PR1 protein levels in vivo . Similar to GT1-7 cells, acute ICV infusion of leptin increased S1PR1 protein levels in the hypothalamus of control rats, as demonstrated in the time-course study ( Fig. 5d ). On the other hand, ICV JSI-124 pretreatment blocked the effect of leptin on hypothalamic S1PR1 protein levels in rats ( Fig. 5e ). To confirm the role of leptin in the control of hypothalamic S1PR1 expression in vivo , we examine the S1PR1 protein content in the hypothalamus of mice lacking leptin ( ob/ob ). Interestingly, ob/ob mice display dramatic reduction on S1PR1 expression (88%) in the hypothalamus, when compared with wild-type mice ( Fig. 5f ). Similar results were found in mice with deficiency in the leptin signalling, db/db mice ( Fig. 5g ). These data demonstrate that STAT3 activation plays a reciprocal role in the regulation of hypothalamic S1PR1 protein levels. Downregulation of hypothalamic S1PR1 in obese rodents Based on our results, we hypothesized that S1PR1 expression could be affected in the hypothalamus under obesity condition, as a reflex of the leptin resistance. Thus, we then examined the effects of high-fat diet (HFD) on hypothalamic leptin resistance and S1PR1 protein levels. Initially, we observed that HFD reduced the hypothalamic S1PR1 protein levels by about 35%, 50% and 75%, in Wistar rats, C57BL6/J and Swiss mice, respectively ( Fig. 6a–c ). Consistent with the S1PR1 protein levels, real-time PCR analysis revealed low S1PR1 mRNA levels in the hypothalamus of Wistar rats after HFD treatment ( Fig. 6d ). 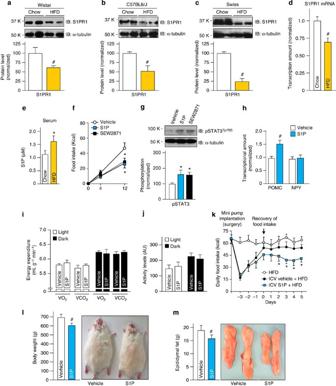Figure 6: Defective S1PR1 expression in the hypothalamus of obese rodents. Western blottings show S1PR1 protein levels in the hypothalamus of (a) Wistar rats (n=8), (b) C57BL6/J mice (n=4) and (c) Swiss mice (n=4) after HFD treatment. (d) Hypothalamic S1PR1 mRNA levels in control and obese Wistar rats (n=10). (e) Determination of S1P serum levels in control and obese C57BL6/J mice (n=6–8). (f) Determination of food consumption after ICV injection of vehicle (dimethylsulphoxide (DMSO)), S1P (50 ng) and SEW2871 (50 nM) in obese rats (n=8). (g) Western blotting shows S1P- and SEW2871-induced STAT3tyr705phosphorylation in hypothalamic samples of obese Wistar rats (n=6). (h) POMC and NPY mRNA were examined using real-time PCR assay 9 h after ICV S1P (50 ng) injection (n=8). (i) Oxygen consumption/carbon dioxide production after single injection of S1P into the third ventricle of obese rats (n=5). (j) Locomotor activity (n=5). (k) Determination of food consumption after chronic ICV infusion of S1P 2.08 ng h−1or vehicle 0.25 μl h−1through the osmotic mini-pump during 9 days. (l) Total body weight and (m) epididymal fat pad weight after chronic delivery of S1P in the hypothalamus of obese rats (n=6). Data were expressed by using mean±s.e.m.#P<0.05 versus chow and *P<0.05 versus obese plus vehicle (Student’st-test). Figure 6: Defective S1PR1 expression in the hypothalamus of obese rodents. Western blottings show S1PR1 protein levels in the hypothalamus of ( a ) Wistar rats ( n =8), ( b ) C57BL6/J mice ( n =4) and ( c ) Swiss mice ( n =4) after HFD treatment. ( d ) Hypothalamic S1PR1 mRNA levels in control and obese Wistar rats ( n =10). ( e ) Determination of S1P serum levels in control and obese C57BL6/J mice ( n =6–8). ( f ) Determination of food consumption after ICV injection of vehicle (dimethylsulphoxide (DMSO)), S1P (50 ng) and SEW2871 (50 nM) in obese rats ( n =8). ( g ) Western blotting shows S1P- and SEW2871-induced STAT3 tyr705 phosphorylation in hypothalamic samples of obese Wistar rats ( n =6). ( h ) POMC and NPY mRNA were examined using real-time PCR assay 9 h after ICV S1P (50 ng) injection ( n =8). ( i ) Oxygen consumption/carbon dioxide production after single injection of S1P into the third ventricle of obese rats ( n =5). ( j ) Locomotor activity ( n =5). ( k ) Determination of food consumption after chronic ICV infusion of S1P 2.08 ng h −1 or vehicle 0.25 μl h −1 through the osmotic mini-pump during 9 days. ( l ) Total body weight and ( m ) epididymal fat pad weight after chronic delivery of S1P in the hypothalamus of obese rats ( n =6). Data were expressed by using mean±s.e.m. # P <0.05 versus chow and * P <0.05 versus obese plus vehicle (Student’s t -test). Full size image We next evaluate the effects of leptin to induce S1PR1 protein levels in the hypothalamus of lean and obese rats. Initially, we observed that ICV infusion of leptin promoted a strong STAT3 tyrosine phosphorylation in control but not in obese animals, as expected ( Supplementary Fig. 3A ). Thereafter, we note that in contrast to lean animal, acute ICV injection of leptin failed to increase S1PR1 mRNA ( Supplementary Fig. 3B ) and protein levels ( Supplementary Fig. 3C ) in the hypothalamus of obese rats. These data demonstrate that central leptin resistance is associated with the downregulation of S1PR1 in the hypothalamus of obese rats. We then monitored the S1P serum levels in obese animals, using ELISA kit specific to detect S1P in the serum of mouse. We observed that obese mice (C57BL6/J) displayed an augment in the serum levels of S1P when compared with control group ( Fig. 6e ). The high levels of S1P suggest that it could be a compensatory mechanism to subvert the downregulation of S1PR1 and defective STAT3 activity in the hypothalamus of obese mice. Thus, we investigated whether the forced activation of S1PR1 in the hypothalamus of obese animals through S1P ICV injection is capable of overcoming leptin resistance, activate STAT3 and recapitulate the anorexigenic signals in obese rats. We performed an acute injection of S1P (50 ng) into the third ventricle of obese rats to evaluate the energy intake and STAT3 phosphorylation. As observed in control animals, S1P was sufficient to reduce the food intake in obese rats ( Fig. 6f ); similar results were found when we used a specific S1PR1 activator, SEW2871 ( Fig. 6f ). Western blotting analysis demonstrated that acute S1P or SEW2871 ICV injections were able to increase STAT3 tyrosine phosphorylation in the hypothalamus of obese rats ( Fig. 6g ). Furthermore, acute S1P injection increased POMC mRNA levels in the hypothalamus of obese rats ( Fig. 6h ). However, we did not observe difference in the energy expenditure after acute S1P ICV injection in obese rats when compared with vehicle group ( Fig. 6i ) and no difference was found in the physical activity pattern ( Fig. 6j ). Apparently, the anorexigenic and thermogenic effects of S1P were more robust in lean than obese animals. Thereafter, to evaluate the impact of chronic S1P administration in obese rats, we performed a chronic micro infusion of S1P (0.25 μl h −1 with 50 ng per day) in the hypothalamus using osmotic mini-pump. We observed that chronic S1P delivery in the hypothalamus promoted reduction on daily food intake ( Fig. 6k ), body weight ( Fig. 6l ) and epididymal fat-pad weight in obese rats ( Fig. 6m ), when compared with vehicle infusion. These data demonstrated that chronic S1P administration into the third ventricle of animals reduced the food consumption and body weight in obese rats. Aberrant S1PR1 activation during cancer-induced anorexia Several studies have demonstrated that S1P levels are involved in persistent STAT3 activation in cancer cells and in tumour microenvironment, and for malignant progression [13] , [14] . In addition, high levels of circulating S1P levels were found in tumour-bearing animals [14] , [30] . In line with these evidences, we sought to investigate whether S1P contributes to anorexia in tumour-bearing rodents. We examined S1PR1 protein levels in the hypothalamus of rats injected with Walker-256 tumour cells and in mice injected with Lewis lung carcinoma (LLC) during tumour-induced anorexia. The LLC cells induced severe anorexia and weight loss in mice ( Fig. 7a–c ). Interestingly, 4 days after onset of anorexia, high levels of S1PR1 protein levels and hyperphosphorylation of STAT3 were found in hypothalamic tissue of anorectic mice ( Fig. 7d ). Despite the high levels of hypothalamic S1PR1 in anorectic mice, we sought to determine the subcellular localization of this receptor. We detected the abundance of S1PR1 in the membrane and cytoplasm in samples obtained from hypothalamus anorectic mice, when compared with control animals ( Supplementary Fig. 3D,E ). 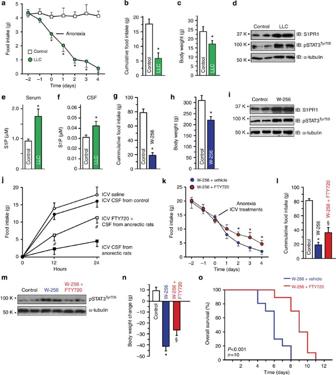Figure 7: Hyperactivation of S1PR1/STAT3 signalling in the hypothalamus during cancer-induced anorexia. (a) Daily food intake determination in C57BL6/J mice injected with LLC (n=6). (b) Cumulative food intake (4 days) after the onset of anorexia in C57BL6/J mice injected with LLC (n=6). (c) Total body weight 4 days after onset of anorexia in mice with LLC cancer, excluding the tumour weight (n=6). (d) Western blotting analysis was performed to evaluate hypothalamic S1PR1 protein level (upper panel) and STAT3 tyrosine phosphorylation (middle panel) in tumour-bearing mice 4 days after the onset of anorexia. (e) S1P serum levels in anorectic mice. These samples were obtained 4 days after the onset of anorexia. (f) CSF levels in control and in anorectic mice. (g) Cumulative food intake (4 days) after the onset of anorexia in Wistar rats (n=8). (h) Total body weight 4 days after onset of anorexia in Wistar rats, excluding the tumour weight (n=8). (i) Western blotting analysis was performed to evaluate hypothalamic S1PR1 protein level (upper panel) and STAT3 tyrosine phosphorylation (middle panel) in tumour-bearing rats 4 days after the onset of anorexia. (j) CSF from control and anorectic rats were injected into the third ventricle of control Wistar rats (2 μl) and then the food consumption was monitored. One group received ICV injection of FTY720 (50 μM) 120 min before the injection of CSF from anorectic rats (n=5). (k) Effects of daily ICV FTY720 (50 nM) injection in tumour-bearing rats on: (k) daily food consumption (n=5), (l) cumulative food intake during 4 days after the onset of anorexia (n=5), (m) STAT3 tyrosine phosphorylation in the hypothalamic tissue (n=4), (n) body weight change (n=5) and (o) survival (n=10). Data were expressed by using mean±s.e.m. *P<0.05 versus respective control group,#P<0.05 versus group injected with CSF from anorectic rats and §P<0.05 versus W-256 group (Student’st-test). The survival curves were estimated using Kaplan–Meier’s estimates, and curves were compared using the log-rank test,P<0.001 (n=10). Figure 7: Hyperactivation of S1PR1/STAT3 signalling in the hypothalamus during cancer-induced anorexia. ( a ) Daily food intake determination in C57BL6/J mice injected with LLC ( n =6). ( b ) Cumulative food intake (4 days) after the onset of anorexia in C57BL6/J mice injected with LLC ( n =6). ( c ) Total body weight 4 days after onset of anorexia in mice with LLC cancer, excluding the tumour weight ( n =6). ( d ) Western blotting analysis was performed to evaluate hypothalamic S1PR1 protein level (upper panel) and STAT3 tyrosine phosphorylation (middle panel) in tumour-bearing mice 4 days after the onset of anorexia. ( e ) S1P serum levels in anorectic mice. These samples were obtained 4 days after the onset of anorexia. ( f ) CSF levels in control and in anorectic mice. ( g ) Cumulative food intake (4 days) after the onset of anorexia in Wistar rats ( n =8). ( h ) Total body weight 4 days after onset of anorexia in Wistar rats, excluding the tumour weight ( n =8). ( i ) Western blotting analysis was performed to evaluate hypothalamic S1PR1 protein level (upper panel) and STAT3 tyrosine phosphorylation (middle panel) in tumour-bearing rats 4 days after the onset of anorexia. ( j ) CSF from control and anorectic rats were injected into the third ventricle of control Wistar rats (2 μl) and then the food consumption was monitored. One group received ICV injection of FTY720 (50 μM) 120 min before the injection of CSF from anorectic rats ( n =5). ( k ) Effects of daily ICV FTY720 (50 nM) injection in tumour-bearing rats on: ( k ) daily food consumption ( n =5), ( l ) cumulative food intake during 4 days after the onset of anorexia ( n =5), ( m ) STAT3 tyrosine phosphorylation in the hypothalamic tissue ( n =4), ( n ) body weight change ( n =5) and ( o ) survival ( n =10). Data were expressed by using mean±s.e.m. * P <0.05 versus respective control group, # P <0.05 versus group injected with CSF from anorectic rats and § P <0.05 versus W-256 group (Student’s t -test). The survival curves were estimated using Kaplan–Meier’s estimates, and curves were compared using the log-rank test, P <0.001 ( n =10). Full size image High S1P serum levels were found in mice during cancer-induced anorexia ( Fig. 7e ). Furthermore, we detected the presence of high levels of S1P in cerebrospinal fluid (CSF) in tumour-bearing mice ( Fig. 7f ), suggesting that S1P could be involved in the aberrant anorexigenic signals in these animals. We also investigate S1PR1 protein level and STAT3 in different models of cancer-induced anorexia. For instance, Walker-256 tumour cells also induced anorexia and weight loss in rats ( Fig. 7g, h ), and high protein levels of S1PR1 and hyperphosphorylation of STAT3 were found in the hypothalamus of anorectic rats with Walker-256 tumour ( Fig. 7i ). To determine whether the presence of S1P in CSF of tumour-bearing animals induces anorexia, we collected CSF from control and anorectic Wistar rats and injected the CSF (2 μl) into the third ventricle of control rats. The acute ICV injection of CSF from control animals did not change the food consumption ( Fig. 7j ); conversely, ICV injection of CSF from anorectic animals promoted a strong anorexigenic effect in control animals ( Fig. 7j ). Interestingly, the anorexigenic effect of CSF from anorectic rats was blunted in animals that received ICV S1PR1 inhibitor (FTY720) pretreatment 60 min before the CSF injection ( Fig. 7j ). To confirm the role of hypothalamic S1PR1 on cancer-induced anorexia, we performed ICV injection of FTY720, a functional antagonist of S1PR1, in Wistar rats during cancer-induced anorexia. FTY720 is an immunosuppressant compound known to modulate the immune system by acting as a functional antagonist of S1PR1 and inducing its internalization and degradation [31] , [32] . After the onset of anorexia, we injected FTY720 (50 μM) daily. Our results revealed that FTY720 increased the daily food consumption ( Fig. 7k ) and cumulative energy intake 4 days after the onset of anorexia ( Fig. 7l ), when compared with vehicle-treated animals. Moreover, FTY720 ICV treatment reduced hypothalamic STAT3 tyrosine phosphorylation in tumour-bearing animals ( Fig. 7m ). This treatment also attenuated cancer-induced weight loss in tumour-bearing rats ( Fig. 7n ). The ICV FTY720 treatment did not change the tumour growth (Tumour+Veh 35.3±2.8 g versus Tumour+FTY720 35.9±3.6 g). Finally, we investigated whether the hypothalamic S1PR1 inhibition increases survival in tumour-bearing animals. After the onset of the anorexia, tumour-bearing animals received a daily ICV injection of vehicle or FTY720 (50 μM). As shown in the Kaplan–Maier graphs, a daily central infusion of FTY720 statistically prolonged the survival in tumour-bearing animals, whereas the median survival of tumour-bearing rats that received vehicle was 6 days and chronic administration of FTY720 increased the median survival to 10 days ( Fig. 7o ). These data suggests that S1P produced during the tumour development triggers hypothalamic anorexigenic signals through the S1PR1/STAT3 axis contributing to cancer-induced anorexia. S1PRs family is composed by five different receptors (1–5) that activate diverse downstream signalling pathways in response to the common S1P [15] . S1PR1 is unique in that it couples exclusively to the G i protein. This receptor is widely expressed, controlling the cellular process in heart, skeletal muscle, colon [14] and other tissues. Although S1P receptors have been identified in the central nervous system [33] , [34] , the presence and function of S1PR1 specifically in the hypothalamus was not reported. Surprisingly, our study revealed that hypothalamic nuclei are highly enriched with S1PR1 protein levels, when compared with peripheral tissues. We identify that S1PR1 is localized in POMC neurons; conversely, low expression of S1PR1 was found in NPY neurons. We also observed that the nutritional availability modulates the hypothalamic S1PR1 expression, whereas under fasting condition hypothalamic S1PR1 protein levels was reduced and refeeding was sufficient to increase S1PR1 in the hypothalamus and this phenomenon was accompanied by STAT3 activity, suggesting the participation of this receptor on the control of the energy homeostasis. The relationship between lysophospholipids and Jak/STAT3 signalling was initially observed in endothelial progenitor cells, once S1P increased Jak2 phosphorylation through the activation of lipid receptor S1PR3 (ref. 35 ); similar results were found in ventricular cardiomyocytes, in this case, S1P increased STAT3 phosphorylation through S1PR2 (ref. 11 ). Although we did not evaluate the presence/function of the others subunits of S1PRs in the hypothalamus, our data revealed that specific S1PR1 activator (SEW2871) promoted consistent STAT3 activation and induced anorexigenic and thermogenic response. However, S1P ICV injection did not change IRS1 tyrosine and Akt serine phosphorylation, suggesting that the effects of S1P/S1PR1 on food intake occurred through the leptin but not insulin signalling. Our data are in accordance with Lee et al . [13] that showed that S1PR1 interacts with Jak2, leading to persistent STAT3 activation in human tumour cells, whereas pharmacological Jak2 inhibitor abrogated S1PR1-mediated STAT3 tyrosine phosphorylation in MB49 tumour cells. We also demonstrated that neuronal S1PR1 induces the anorexigenic signals through the melanocortin system. Importantly, our experimental findings were confirmed by the transcriptome analysis, using the BXD database that displayed a strong correlation among S1PR1 and anorexigenic and thermogenic pathways. This bioinformatic study was able to detect a negative correlation between the hypothalamic S1PR1 levels and the food consumption and body weight in several strains of BXD mice. Using in vivo and in vitro models we observed that leptin increased S1PR1 protein levels in GT1-7 neuronal cells and in the hypothalamus of rats. Importantly, we demonstrated that STAT3 inhibition blunted leptin-induced S1PR1 protein levels in both models. These data could be explained once STAT3 directly binds to and activates the S1pr1 promoter [13] . In addition, our results revealed that leptin deficiency or leptin receptor deficiency lead a strong reduction in S1PR1 hypothalamic levels, as observed in ob/ob and db/db mice. Furthermore, HFD treatment induced central leptin resistance and this phenomenon was accompanied by low hypothalamic S1PR1 protein levels, showing the reciprocal requirement among S1PR1 and STAT3 in hypothalamic neurons. In the present study, the role of S1PR in MBH in the control of the energy balance was investigated using the acute S1PR1 siRNA injection in vivo . This methodology induced the transient S1PR1 downregulation in MBH of mice, promoting consistent hyperphagia and abnormal thermogenic response. Although our data demonstrated that downregulation of S1PR1 protein levels in MBH affect the energy balance, this methodological approach failed to demonstrate the significant difference in the body weight gain of mice. Thus, the role of long-term S1PR1 downregulation in the MBH in the control of the body weight remains unclear and deserves further investigations. Circulating molecules able to activate Jak2/STAT3 in hypothalamic neurons through the cross-talk mechanisms generally affects food intake and energy expenditure in mammals [4] , [5] , [6] , [36] . It has been proposed that alternative activation of Jak2/STAT3 in the hypothalamus through the glycoprotein 130 receptor (gp130R) ligands, for instance, may play as potential therapeutic targets in obesity [37] . Our study provide substantial evidences that a circulating bioactive lipid metabolite, S1P, could be considered the alternative molecule capable to activate Jak2/STAT3 signalling pathway and recapitulate the anorexigenic signals in the hypothalamus. We demonstrated that even with low expression of hypothalamic S1PR1 observed in obese rats, ICV injection of S1P or SEW2871 was sufficient to activate STAT3 and induce anorexigenic effects in obese animals. On the other hand, we detect augment of S1P serum levels in obese mice, when compared with the lean group. These data are in accordance with previous study that demonstrated that plasma levels of S1P were increased in ob/ob mice [38] . The augment in S1P levels in obese mice may occur as a compensatory mechanism despite the low hypothalamic S1PR1levels. However, the increased S1P levels observed in obese animals is not enough to activate the S1PR1/STAT3 signalling in the hypothalamus. The downregulation of S1PR1 protein level in obese rodents seems to be associated with the impairment of central S1P anorexigenic and thermogenic action in obese animals, when compared with lean ones. In addition, the molecular mechanisms of leptin resistance, such as, the protein tyrosine phosphatase 1B [39] , [40] , [41] and IKKβ [42] , [43] , [44] activation may contribute to the impairment of S1PR1/Jak2 association and STAT3 activation in response to S1P; however, this issue deserves further investigations. Using the osmotic mini-pump to delivery S1P specifically in the hypothalamus of obese rats resulted in a significant reduction in food intake and body weight. The S1P synthesis occurs by phosphorylation of sphingosine, in a reaction catalysed by sphingosine kinases, SPHK1 and SPHK2 (ref. 15 ). Although, high levels of S1P were found in obese and in tumour-bearing mice, the S1P sources are distinct in each situation. An elegant study demonstrated in model of colitis-associated cancer in mice that S1P is produced by upregulation of SPHK1 in cancer cells [14] . However, in the obesity state the cell types that promote the S1P synthesis remain unknown. Anorexic cancer patients often report early satiety, which together with a reduced appetite has been postulated to be caused by the production of factors by the tumour that exerts their effects by acting on hypothalamic cells, amplifying the anorexigenic signals [45] , [46] . The pro-inflammatory cytokines such as tumour necrosis factor-α, interleukin 1β and interferon gamma are the major products secreted by the tumour proposed to play a role in the aetiology of cancer-induced anorexia [45] . Studies have reported that aberrant S1P serum levels were found in animal models of cancer [14] , [30] . Moreover, serum levels of S1P were inversely correlated with chemotherapy-induced weight gain in women with breast cancer [47] . During the tumour development, high levels of S1P are produced through the upregulation of SPHK1 activity in cancer cells [14] . In addition, it has been proposed that serum S1P elevation represents the communication between cancer cells and host organism [48] . In our study, high serum and CSF S1P levels were found in tumour-bearing rats and it was associated with the upregulation of S1PR1 protein levels and STAT3 phosphorylation in the hypothalamus. In addition, intraperitoneal injection of S1P induced anorexigenic and thermogenic effects. Interestingly, the disruption of S1P/S1PR1 signalling in the hypothalamus reversed the anorexia in tumour-bearing animals and prolonged the survival in these animals. We suggested that in the late-stage of cancer, S1P produced by cancer or stromal cells acts in the hypothalamus, contributing to cancer-induced anorexia. Taken together, our study shows that neuronal S1P/S1PR1 axis affects the energy homeostasis through the Jak/STAT signalling and melanocortin system in rodents. We determine that S1PR1 and STAT3 play reciprocal effects in the hypothalamus. We also report that neuronal S1P/S1PR1/STAT3 signalling plays an important role in distinct conditions of abnormal feeding behaviour, such as obesity or cancer-induced anorexia. Thus, S1P/S1PR1 axis plays a critical role in the energy balance and represents a potential target for the treatment of obesity and cancer-induced anorexia as well. Animals Wistar rats, Swiss, C57BL/6J, ob/ob and db/db mice were obtained from the University of Campinas Breeding Center. The investigation was approved by the ethics committee of the University of Campinas (CEUA) and followed the university guidelines for the use of animals in experimental studies and experiments conform to the Guide for the Care and Use of Laboratory Animals, published by the U.S. National Institutes of Health (NIH publication number 85-23 revised 1996). Male, 5-week-old Wistar rats and 10-week-old Swiss mice were obtained from the University of Campinas Breeding Center. The animals were maintained in 12 h:12 h artificial light–dark cycles, with lights on at 0600, h, and were housed in individual cages. The animals were randomly divided into two groups: control, fed on standard rodent chow (3.948 kcal h kg −1 ) or HFD (5.358 kcal kg −1 ) ad libitum for 3 months. Male (10-week-old) ob/ob and db/db mice and their respective control C57BL/6J background mice were obtained from The Jackson Laboratory (Bar Harbor, ME). The mice were bred under specific pathogen-free conditions at the Central Breeding Center of the University of Campinas and were fed on standard rodent chow. The number of animals used in each experiment is specified in the legend figure. Antibodies and chemicals Anti-EDG-1 (rabbit polyclonal, SC-25489), Anti-Jak2 (rabbit polyclonal, SC-278), anti-STAT3 (rabbit polyclonal, SC-483), anti-phospho-IRS-1 (rabbit polyclonal, SC-17199), anti-NPY (goat polyclonal, SC-14728) and anti-POMC (rabbit polyclonal, SC-20148) antibodies were from Santa Cruz Biotechnology, Inc. Anti-phospho-Akt (rabbit polyclonal, 9271s), anti-α tubulin (rabbit polyclonal, 2144), anti-phospho-STAT3 (rabbit polyclonal, 9131) and anti-phospho-Jak2 (rabbit polyclonal, 3771) was from Cell Signalling Technology (Beverly, MA, USA). The antibody solution was 1:1,000 for the western blottings and 1:200 for the immunohistochemistry experiments. Leptin was from Calbiochem (San Diego, CA, USA). Protein A-Sepharose 6 MB and nitrocellulose paper (Hybond ECL, 0.45 mm) were from Amersham Pharmacia Biotech United Kingdom Ltd (Buckinghamshire, UK). S1P was from Avanti Polar Lipids Inc. (Alabama, EUA). SEW2871 was from Cayman Chemical (Michigan, USA), FTY720 was from Cayman Chemical Company (Michigan, USA) and Cucurbitacin JSI 124 was from Sigma Chemical Co. (St Louis, MO). SHU9119 was from Tocris Bioscience (Bristol, UK). Routine reagents were purchased from Sigma Chemical Co. (St Louis, MO) unless otherwise specified. Determination of S1P levels After 6 h of fasting, blood was collected from the cava vein. Plasma was separated by centrifugation (1,100 g ) for 15 min at 4 °C and stored at −80 °C until the assay. CSF was obtained from male rats through the cisterna magna puncture using the stereotaxic apparatus. For serum and CSF S1P determination, we employed a commercially available Sphingosine-1 phosphate Assay kit (Echelon Biosciences Inc.). Cell culture The mouse hypothalamic tumour cell line GT1-7 were obtained from the laboratory of Dr Pamela Mellon, San Diego, CA, USA [49] . GT1-7 cells were cultured in DMEM medium containing 10% of fetal bovine serum (FBS), with the addition of antibiotics and fungicides in a humid atmosphere with 37 °C, 5% CO 2 . The LLC cells were obtained from ATCC, Philadelphia, PA, USA, and the Walker-256 tumour cell line (originally obtained from the Christ Hospital Line, National Cancer Institute Bank, Cambridge, UK). Cells were cultured in RPMI containing 10% FBS and glutamine without addition of antibiotics or fungicides; they were maintained at 37 °C, 5% CO 2 . In vitro and in vivo siRNAs transfection For in vitro study, a total of 5 × 10 5 cells were seeded in a tissue culture plate in complete growth medium and incubated overnight. Transfection with siRNA targeted to STAT3 (si-STAT3 Silencer Select Pre-designed s744) or scrambled control siRNA (Silencer Select Pre-designed 4309843) was performed. GT1-7 cells were washed twice with serum- and glucose-free medium (Opti-MEM, Life Technologies, Gaithersburg, MD, USA) and then incubated with 2 ml of the same medium containing the siRNA (final concentration of 100 nM) previously mixed with 5 μl of Lipofectamine 2000 (Life Technologies). After 7 h, 1 ml of Opti-MEM medium containing 30% FBS was added to the culture containing siRNAs and Lipofectamine. After 17 h, cells were cultured in DMEM medium with 10% of FBS for 12 h. After this period, cells were starved overnight and treated with leptin (40 μmol l −1 ) for 12 h. Subsequently, the cells were used for western blot analysis. For the in vivo study, we used jetSI 10 mM S1PR1 siRNA specifc for rodent brain. The Invivofectamine 2.0 Reagent (Invitrogen, CA, USA) was mixed with the siRNA targeted to S1PR1 (Silencer Select Pre-designed s65290) or the negative control (Silencer Select Negative Control si RNA, in vivo ready), according to the manufacturer’s instructions. The siRNA plus invivofectamine solution (4 μl, 1 mg ml −1 ) was carefully injected and the experiments were carried out within 72 h. Tumour xenograft models Male C57BL6/J mice were implanted with 1.0 × 10 6 LLC into the dorsal subcutis of the right flank. Four days after the onset of anorexia, mice were killed, the hypothalamic tissue was excised and mice were weighed with and without tumour. Walker-256 tumour cells were obtained from the ascitic fluid of the peritoneal cavity of Wistar rats 5 days after the intraperitoneal injection of 20 × 10 6 carcinoma cells. After cell harvesting, the percentage of viable cells was determined by using 1% Trypan blue solution in a Neubauer chamber. Tumour cells (2 × 10 6 cells in 1 ml saline solution) were injected in the right flank after the surgical implantation of the ICV cannula. Definition of cancer anorexia Each animal’s individual baseline 24-h food intake was defined as the average daily food intake over a period of 3 consecutive days. Subsequent food intake data are expressed as individual percentages and baseline daily food intake. In tumour-bearing animals, cancer anorexia was defined as a single value of <70% of baseline occurring after a steady decline of at least 3 days duration. Intracerebroventricular cannulation After intraperitoneal injection of a mixture of ketamin (10 mg) and diazepam (0.07 mg; 0.2 ml per 100 g body weight), male Wistar rats (12-week-old) were stereotaxically instrumented with a chronic 26-gauge stainless steel indwelling guide cannula aseptically placed into the third ventricle at the midline coordinates of 0.5 mm posterior to the bregma and 8.5 mm below the surface of the skull of the rats using the Stoelting stereotaxic apparatus. The VMH of rats was accessed bilaterally using a 25-gauge needle connected to Hamilton 25 μl syringes. VMH and MBH S1P injections The vehicle and S1P injections in rats were directed to stereotaxic coordinates 2.3/3.3 mm posterior to the bregma, ±0.6 mm lateral to midline and 10.2 mm below the surface of the skull [18] . In mice, the MBH injections were made using the coordinates, as previously published by Zhang et al . [44] Intracerebroventricular injections Rats were deprived of food for 2 h with free access to water and received 2 μl of bolus injections into the third ventricle, as follows: Leptin injection . Rats received ICV infusion of vehicle (saline) or leptin (10 −6 M) at 1800, h to evaluate the food consumption. Food intake was determined by measuring the difference between the weight of chow given and the weight of chow at the end of a 4- and 12-h period. To evaluate the effects of leptin on Jak/STAT signalling, the hypothalamic tissue was removed 30 min later. To evaluate the effects of leptin on S1PR1 protein levels, the hypothalamic tissue was removed 8 and 12 h after leptin ICV injection. Sphingosine-1 phosphate . For western blot analysis, ICV S1P (2 and 50 ng) was injected into the third ventricle. To evaluate the effects of S1P on Jak/STAT signalling, the hypothalamic tissue was removed 30 min later. To evaluate the effects of S1P on food intake in rats, ICV injection of S1P (50 ng) was performed at 1800, h. SEW2871 . For western blot analysis, ICV SEW2871 (50 nM) was injected into the third ventricle. To evaluate the effects of SEW2871 on STAT3 phosphorylation, the hypothalamic tissue was removed 30 min later. To evaluate the effects of SEW2871 on food intake in rats, ICV injection of S1P (50 ng) was performed at 1800, h. JSI124 . For western blot analysis, ICV JSI124 (50 μM) was injected into the third ventricle. To evaluate the effects of JSI124 on STAT3 phosphorylation, the hypothalamic tissue was removed 60 min later. To evaluate the effects of JSI124 on food intake in rats, ICV JSI124 injection was performed 30 min before the S1P injection. FTY720 . To evaluate the effects of FTY720 on food intake in tumour-bearing rats, daily ICV injections (50 μM) was performed at 1800, h. Thirty minutes after the last injection, the hypothalamic tissue was removed for western blotting analysis. SHU9119 . To evaluate the effects of S1P on melanocortin system, ICV of SHU9119 (1 mmol) was performed 30 min before the S1P injection. Thereafter, the food consumption was monitored 4 and 12 h later. Cerebrospinal fluid injection . CSF from control or from tumour-bearing Wistar rats were obtained through the introduction of a needle into the cisterna magna through the skin and/or dura mater using a stereotactic micromanipulator. Immediately after the liquor sampling, 2 μl were injected into the third ventricle of control rats to evaluate the food intake. One group of rats received ICV injection of FTY720 (50 μM) 120 min before the CSF injection. CSF injections were performed at 1800, h. Mini pump For chronic S1P ICV administration, obese rats were submitted to ICV cannulae, which were implanted under ketamin and diazepam as described above. A catheter tube was connected from the brain infusion cannulae to a mini-osmotic pump (model 2002, Alzet, DURECT Corporation, Cupertino, CA) infusing 2.08 ng h −1 of S1P (50 ng within 24 h) or vehicle 0.25 μl h −1 . A subcutaneous incision on the dorsal surface of the animal was created where the pump was inserted. Intraperitoneal S1P injection Single intraperitoneal S1P (100 ng) or vehicle injection was performed in C57BL6/J lean mice. These injections were performed at 1800, h, and then food consumption and oxygen consumption/carbon dioxide production were measured in LE405 Gas Analyzer (Panlab—Harvard Apparatus, Holliston, MA, USA). Core temperature measurement An incision was performed in lateral abdominal wall of animals to insert in the peritoneal cavity the temperature datalogger probe (Subcue Dataloggers, Calgary, AB, Canada). After the surgical wound was sutured in layers, the animals were recovered from surgery at least 5 days before experimental protocol. The probe was programmed to acquire data every 15 min. Oxygen consumption and locomotor activity determination Oxygen consumption and carbon dioxide production were measured in fed animals through a computer-controlled, open circuit calorimeter system LE405 Gas Analyzer (Panlab—Harvard Apparatus). Animals were singly housed in clear respiratory chambers and room air was passed through chambers at a flow rate of ten times the respective weight of each animal. The air flow within each chamber was monitored by a sensor Air Supply & Switching (Panlab—Harvard Apparatus). Gas sensors were calibrated before the onset of experiments with primary gas standards containing known concentrations of O 2 , CO 2 and N 2 (Air Liquid, Sao Paulo, Brazil). The analyses were performed in triplicates of 6 min for each chamber. Therefore, each animal was evaluated for 24 h. Outdoor air reference values were sampled after every four measurements. Sample air was sequentially passed through O 2 and CO 2 sensors to determine O 2 and CO 2 content, from which measures of oxygen consumption (VO 2 ) and carbon dioxide production (VCO 2 ) were estimated. The VO 2 and VCO 2 were calculated by Metabolism 2.2v software and expressed in ml g −1 min −1 , based on Withers equation. The spontaneous locomotor activity was evaluated over a 24-h period using a computer-controlled detection system from Panlab—Harvard Apparatus. Taste reactivity test The video cameras were placed outside the chamber, 300 mm from the ring holding the food cup. After S1P ICV injection, the animal behaviours were monitored during 15 min. The video signal was recorded at 50 frames per second. The videos were analysed by slow-motion playback to count taste reactivity components. Taste reactivity components were classified as hedonic, aversive, or neutral, as previously determined. Immunohistochemistry Paraformaldehyde-fixed hypothalami were sectioned (5 μm). The sections were obtained from the hypothalami of five rats per group in the same localization (antero–posterior=−1.78 from bregma) and were subjected to regular single- or double-immunofluorescence staining using 4',6-diamidino-2-phenylindole, anti-S1PR1, anti-POMC, anti-NPY, anti-STAT3 and anti-glial fibrillary acidic protein antibodies. Analysis and photodocumentation of results were performed using a LSM 510 laser confocal microscope (Zeiss, Jena, Germany). The anatomical correlations were made according to the landmarks given in a stereotaxic atlas. Dissection of the hypothalamic regions Hypothalamic nuclei of rats were quickly dissected in a stainless steel matrix with razor blades and frozen in liquid nitrogen. Later on, each region of the hypothalamus was dissected from 1-mm-thick sagittal sections of fresh brain. PVN, Arc and VMH plus DMH were dissected from the first sections from the midline of the brain. Coordinates for each hypothalamic region are as follows; PVN: square area with anterior margin (posterior region of anterior commisure), dorsal margin (border with thalamus), ventral margin and posterior margin (white matter separating PVN/anterior hypothalamus and VMH/DMH); VMH plus DMH: triangular area with anterior margin (white matter separating PVN/anterior hypothalamus and VMH/DMH), posterior margin (border with mammilary body) and ventral margin (border with Arc); Arc: ventral part of the medial hypothalamus with anterior and dorsal margin and posterior margin (border with mammilary body). mRNA isolation and real-time PCR Hypothalamic total RNA was extracted using Trizol reagent (Life Technologies), according to the manufacturer’s recommendations. Total RNA was rendered genomic DNA free by digestion with Rnase-free Dnase (RQ1, Promega, Madison, WI, USA). Rats were deprived of food for 9 h for real-time PCR analysis. Real-time PCR and mRNA isolation were performed using a commercial kit, as follows: POMC: Rn00595020_m1, NPY: Rn00561681_m1, GAPD, 4352338E, S1PR1: Rn.PT.56a.12493708 for rat and RPS-29 (NCBI: NM012876), sense: 59- AGGCAAGATGGGTCACCAGC -39, antisense: 59- AGTCGAATCATCCATTCAGGTCfG -39. Subcellular fractionation The hypothalamus from rats were homogenized in 2 volumes of STE buffer (0.32 M sucrose, 20 mM Tris·HCl (pH 7.4), 2 mM EDTA, 1 mM dithiothreitol, 100 mM sodium fluoride, 100 mM sodium pyrophosphate, 10 mM sodium orthovanadate, 1 mM phenylmethylsulphonyl fluoride (PMSF) and 0.1 mg aprotinin per ml) at 4 °C. The homogenates were centrifuged (1,000 g , 25 min, 4 °C) to obtain pellets. The pellets were washed once with STE buffer (1.000 g, 10 min, 4 °C) and suspended in Triton buffer (1% Triton X-100, 20 mM Tris HCl (pH 7.4), 150 mM NaCl, 200 mM EDTA, 10 mM sodium orthovanadate, 1 mM PMSF, 100 mM NaF, 100 mM sodium pyrophosphate and 0.1 mg aprotinin per ml), kept on ice for 30 min and centrifuged (15,000 g , 30 min, 4 °C) to obtain the nuclear fraction. The supernatant was centrifuged (100,000 g , 60 min, 4 °C) to obtain the cytosol fraction and the pellet, which was suspended in STE buffer+1% NP-40, kept on ice for 20 min and centrifuged (100,000 g , 20 min) to obtain the membrane fraction. The fractions were treated with Laemmli buffer with 100 mM dithiothreitol and heated in a boiling water bath for 5 min, and aliquots (0.2 mg of protein) were subjected to western blotting analysis. Western blotting analysis and immunoprecipitation The animals were anaesthetized, and the hypothalamus, cerebellum, midbrain, cortex, liver, heart, gastrocnemius muscle and adipose tissue were quickly removed, minced coarsely and homogenized immediately in a freshly prepared ice-cold buffer (1% Triton X-100, 100 mmol l −1 Tris pH 7.4, 100 mmol l −1 sodium pyrophosphate, 100 mmol l −1 sodium fluoride, 10 mmol l −1 EDTA, 10 mmol l −1 sodium vanadate, 2 mmol l −1 phenylPMSF and 0.1 mg aprotinin) suitable for preserving the phosphorylation states of enzymes. Jak2 was immunoprecipitated from rat hypothalami. Antibodies used for immunoblotting were anti-S1PR1 and anti-Jak2. Blots were exposed to preflashed Kodak XAR film. Band intensities were quantified by optical densitometry (UN-SCAN-IT gel, 6.1) of the developed autoradiographs. Uncropped images of Western blots are shown in Supplementary Fig. 4 . Bioinformatics analysis Correlation analyses were performed using hypothalamic mRNAs of BXD inbred family (Hypothalamus Affy MoGene 1.0 ST (Nov10)) and are accessible on Genetwork ( http://www.genenetwork.org ) and NCBI GEO (GSE36674, http://www.ncbi.nlm.nih.gov/geo ) as described in (PMID: 22939713). Correlation matrix graph was built using corrgram package in R ( http://www.r-project.org ). The values used are available in the Supplementary Tables 1 and 2 . Statistical analysis All numeric results are expressed as the means±s.e.m. of the indicated number of experiments. The results of blots are presented as direct comparisons of bands in autoradiographs and quantified by optical densitometry (UN-SCAN-IT gel, 6.1). Statistical analysis was performed using the Student’s t -test and analysis of variance test with the Bonferroni post test. Significance was established at the P <0.05 level. The survival curves were estimated using Kaplan–Meier’s estimates, and curves were compared using the log-rank test and the level of significance was set at P <0.001. How to cite this article: Silva, V.R.R et al . Hypothalamic S1P/S1PR1 axis controls energy homeostasis. Nat. Commun. 5:4859 doi: 10.1038/ncomms5859 (2014).